ptk7mutant zebrafish models of congenital and idiopathic scoliosis implicate dysregulated Wnt signalling in disease Scoliosis is a complex genetic disorder of the musculoskeletal system, characterized by three-dimensional rotation of the spine. Curvatures caused by malformed vertebrae (congenital scoliosis (CS)) are apparent at birth. Spinal curvatures with no underlying vertebral abnormality (idiopathic scoliosis (IS)) most commonly manifest during adolescence. The genetic and biological mechanisms responsible for IS remain poorly understood due largely to limited experimental models. Here we describe zygotic ptk7 (Z ptk7 ) mutant zebrafish, deficient in a critical regulator of Wnt signalling, as the first genetically defined developmental model of IS. We identify a novel sequence variant within a single IS patient that disrupts PTK7 function, consistent with a role for dysregulated Wnt activity in disease pathogenesis. Furthermore, we demonstrate that embryonic loss-of-gene function in maternal-zygotic ptk7 mutants (MZ ptk7 ) leads to vertebral anomalies associated with CS. Our data suggest novel molecular origins of, and genetic links between, congenital and idiopathic forms of disease. Scoliosis refers to spinal curvature >10 degrees and can occur as a consequence of vertebral malformations, underlying congenital or juvenile disease, or with no identifiable primary cause [1] , [2] . Scoliosis caused by congenital vertebral malformation (CVM) is referred to as congenital scoliosis (CS) and affects 0.13–0.5 of 1,000 live human births [1] , [3] . CVMs like hemivertebrae, wedge-shaped vertebrae, vertebral fusions and/or vertebral bar can exist throughout the spine and often impose severe deformity on affected individuals. In mammals, vertebral bodies are derived from somites—periodic segments of paraxial mesoderm that form in pairs along the cranial-to-caudal axis in response to an internal ‘segmentation clock’. Briefly, a molecular network of Notch, canonical Wnt/β-catenin and FGF signalling pathways generate travelling waves of gene expression along the posterior body axis that drive rhythmic somite production from the presomitic mesoderm (PSM) (reviewed in ref. 4 ). To date, most mutations associated with human CS disrupt Notch segmentation genes [5] , [6] , [7] , [8] , [9] . However, the genetic basis of the majority of CVMs remains unknown. The most prevalent forms of human spinal curvature are idiopathic (that is, with no underlying pathology). Idiopathic scoliosis (IS) affects ~3% of children worldwide, with many individuals eventually requiring some form of clinical intervention [1] , [10] . IS typically presents during adolescence as a three-dimensional rotation of the spine that has a propensity to increase in magnitude up to sexual maturity. These deformities range in both severity and progression with a significant bias for severe curves in females [11] , [12] . Familial clustering and concordance among monozygotic twins indicates a primary genetic cause for IS (refs 13 , 14 ) and genome-wide association studies have identified polymorphisms associated with IS in divergent human populations [15] , [16] , [17] . However, phenotypic and genetic heterogeneity have typically made it difficult to define causative mutations in humans. Limitations inherent to the available developmental and genetic animal models of scoliosis have slowed our basic understanding of IS pathogenesis [18] , [19] . Fundamentally, scoliosis does not readily develop in most laboratory animals and induction of IS-like deformities requires drastic surgical or systemic interventions that preclude relevance to human disease [18] . Rodents are quadrupeds and the structure of their spine and centre of gravity are quite different from humans. Tellingly, rodents only become susceptible to spinal curves when forced to walk upright [20] , [21] , revealing the importance of biomechanics and spinal loading during IS progression. Bipedalism has made induced chick models popular; however, in chick, anatomical restraints on spinal mobility are likely protective and prevent the full range of spinal curvatures that can develop in humans [22] . In contrast, spinal deformity is naturally common among teleosts, with nutritional, environmental and/or genetic factors associated with curvature in different species and fish populations [12] , [23] . Teleosts experience cranial-to-caudal spinal loads (similar to humans) that are generated as a function of swimming forward through dense media/water coupled with caudal tail-propulsion. Thus, similar biomechanical forces along the spine may make fish more susceptible to late-onset spinal curvatures [12] . Interestingly, heritable scoliosis-like phenotypes have been characterized in fish raising the intriguing possibility that teleosts can effectively model human IS [12] , [23] . However, the genetic lesions responsible for late-onset spinal curvatures in these fish models have not yet been identified. We have previously reported the generation of protein tyrosine kinase 7 ( ptk7 ) mutant zebrafish ( ptk7a , Ensembl Zv9; ref. 24 ). Ptk7 is an evolutionarily conserved atypical receptor tyrosine kinase that has been implicated in vertebrate Wnt, Semaphorin/Plexin and VEGF signal transduction [24] , [25] , [26] , [27] , [28] , [29] , [30] . Our analysis of patterning and morphogenesis defects in maternal-zygotic ptk7 mutant embryos (MZ ptk7 ), which demonstrate early and complete loss-of-gene function, revealed essential roles for Ptk7 in regulating multiple branches of Wnt signal transduction [24] . Specifically, we demonstrated a key role for Ptk7 in potentiating non-canonical Wnt/planar cell polarity (PCP) signals that coordinate polarized cell movements to shape the body axis during gastrulation and neurulation [31] , as well as negatively regulating canonical Wnt/β-catenin activity [24] . Remarkably, embryonic defects are fully rescued in Z ptk7 mutant embryos, highlighting an important role for early maternal gene function in developmental patterning and morphogenesis. In this study we characterize Z ptk7 and MZ ptk7 mutant zebrafish as functional models of idiopathic and congenital scoliosis, respectively. We demonstrate that zygotic ptk7 mutant fish display fully penetrant late-onset spinal curvature that is not associated with vertebral malformations, is sexually dimorphic and variable in both time of onset and severity. Our work thus establishes Z ptk7 mutant zebrafish as the first genetically defined developmental model of human IS. Moreover, we demonstrate that a novel PTK7 mutation identified in a single human IS patient disrupts both PCP and Wnt/β-catenin signalling, further suggesting that dysregulated Wnt activity may contribute to disease. Conversely, early loss of Ptk7 function in MZ ptk7 mutant larvae results in CS-like vertebral malformations. These CVMs may be attributed to earlier defects in segmentation caused by PCP and Wnt/β-catenin signalling defects. Together, our data suggests a genetic link between CS and IS and highlights the utility of zebrafish for modelling human spinal deformities. Z ptk7 mutants develop late-onset spinal curves that model IS Z ptk7 mutant embryos do not show defects in embryonic patterning or morphogenesis, as maternal Ptk7 is sufficient to rescue early development [24] . However, at late larval and early juvenile stages, all Z ptk7 mutant fish develop scoliosis with spinal curvatures of variable magnitude observed in both the sagittal and coronal axes ( Fig. 1a,b ). In zebrafish, spinal deformities can often be caused by Pseudolomoa neurophilia , Aeromonas hydrophila , and mycobacterium spp. infection. To determine whether observed scoliosis was secondary to an infectious agent, Z ptk7 mutant fish with severe spinal curvatures were sent to the Zebrafish International Resource Center Health Services (Eugene, Oregon) for histopathology. All samples tested negative for infection, indicating a more direct link between ptk7 mutation and spinal curve development. 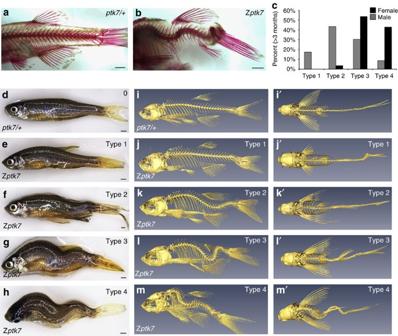Figure 1: Zygoticptk7mutants display late-onset, three-dimensional spinal curvatures. (a,b) Lateral views of trunk and tail skeleton stained with alizarin red for (a)ptk7/+and (b) zygoticptk7(Zptk7) mutant male zebrafish at ~6 months of age. Scale bars, 1 mm. (c) Graph depicting phenotypic and gender distributions for type 1–4 classification based on curve severity at sexual maturity (~3 months of age). Quantification is represented as a percentage of the total for male (n=92) and female (n=58) zebrafish. (d–h) Adultptk7/+and Zptk7mutant zebrafish representative of each curve severity class: (d) unaffectedptk7heterozygote zebrafish (type 0); (e) mild curvature (type 1); (f) moderate curvature (type 2) primarily isolated to the tail; (g) progressed curvature (type 3) with trunk, tail and mild medio-lateral rotations; (h) severe curvature (type 4) with extreme trunk, tail and medio-lateral rotations. Scale bars, 1 mm. (i–m) Lateral and (i′–m′) dorsal views of three-dimensional microCT renderings of adult (i)ptk7heterozygote as well as (j) type 1, (k) type 2, (l) type 3 and (m) type 4 Zptk7mutant zebrafish. Figure 1: Zygotic ptk7 mutants display late-onset, three-dimensional spinal curvatures. ( a , b ) Lateral views of trunk and tail skeleton stained with alizarin red for ( a ) ptk7/+ and ( b ) zygotic ptk7 (Z ptk7 ) mutant male zebrafish at ~6 months of age. Scale bars, 1 mm. ( c ) Graph depicting phenotypic and gender distributions for type 1–4 classification based on curve severity at sexual maturity (~3 months of age). Quantification is represented as a percentage of the total for male ( n =92) and female ( n =58) zebrafish. ( d – h ) Adult ptk7/+ and Z ptk7 mutant zebrafish representative of each curve severity class: ( d ) unaffected ptk7 heterozygote zebrafish (type 0); ( e ) mild curvature (type 1); ( f ) moderate curvature (type 2) primarily isolated to the tail; ( g ) progressed curvature (type 3) with trunk, tail and mild medio-lateral rotations; ( h ) severe curvature (type 4) with extreme trunk, tail and medio-lateral rotations. Scale bars, 1 mm. ( i – m ) Lateral and ( i′ – m′ ) dorsal views of three-dimensional microCT renderings of adult ( i ) ptk7 heterozygote as well as ( j ) type 1, ( k ) type 2, ( l ) type 3 and ( m ) type 4 Z ptk7 mutant zebrafish. Full size image To determine whether observed scoliosis resulted from CVMs, vertebrae formation was imaged in Z ptk7 mutant and control animals using calcein stain (a vital, fluorescent calcium-binding chromophore) [32] . Larvae were analyzed at 4, 4.5 and 6.0 mm standard length. No defects in vertebral patterning or formation were observed in Z ptk7 mutants ( n =33) compared with ptk7 /+ siblings ( n =40; Fig. 2a–f ). High-resolution micron-scale computed tomography (microCT) was then performed to further examine spinal curvature and vertebral structure in Z ptk7 mutant zebrafish. Three-dimensional skeletal reconstructions of 12 Z ptk7 mutant adults and 3 ptk7/+ siblings revealed the profound late-onset curvatures typical of mutant fish and confirmed that abnormal vertebral patterning is not a general aspect of the Z ptk7 mutant phenotype ( Fig. 1i,m ; Supplementary Movies 1–5 ). 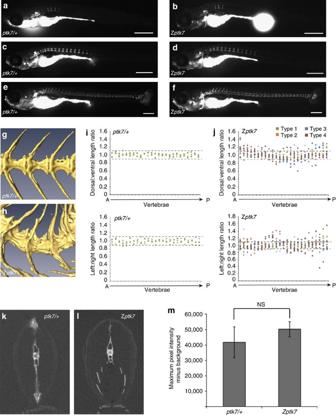Figure 2: Zygoticptk7mutants do not display vertebral patterning abnormalities but do show vertebral ‘wedging’ reminiscent of human IS. (a–f) Live calcein staining of (a,b) 4 mm, (c,d) 4.5 mm and (e,f) 6.0 mm (a,c,e)ptk7heterozygote and (b,d,f) zygoticptk7(Zptk7) mutant larvae. All scale bars, 0.5 mm. (g,h) Lateral views of caudal vertebrae from three-dimensional microCT renderings of adult (g)ptk7heterozygote and (h) Zptk7mutant zebrafish.Ptk7mutant vertebrae display a wedge-shaped morphology at the apex of curves. (i,j) Graphs depicting dorsal:ventral and left:right length ratios of trunk and tail vertebrae inptk7heterozygote (i;n=3) and Zptk7mutant (j;n=12) zebrafish. To characterize vertebral shape changes, we measured the length of individual thoracic and tail vertebrae along the dorsal, ventral, left and right sides. We calculated dorsal:ventral and left:right length ratios to assess possible length asymmetries in the dorso-ventral and medio-lateral planes, respectively. Horizontal dotted lines demarcate arbitrary±0.1, determined by the maximum deviation from 1 inptk7heterozygote controls and used to illustrate the deviation of Zptk7vertebrae from normal. Deviation from 1±0.1 is evident at multiple vertebrae in three dimensions along the entire length of the spine. Type 1–4 Zptk7mutants are grouped by point colour, and each individual fish is represented by a unique point shape and colour. The graph’s horizontal axis spans anterior (A) to posterior (P), from the first abdominal vertebrae to the last caudal vertebrae. The Weberian and caudal tail vertebrae were excluded from our analysis. (k,l) Maximum intensity projections (MIP) in the cranio–caudal direction from high-resolution micro-computed tomography (microCT) of (k)ptk7/+ and (l) Zptk7mutant zebrafish. Dorsal is up and ventral is down. (m) Quantification of maximum pixel intensity corrected for background intensity to infer approximate bone density inptk7/+ (n=3) and Zptk7(n=12) zebrafish. Maximum pixel intensities of the vertebrae were extracted from MIPs made from 10 sequential microCT slices. Three locations from trunk to tail were quantified and averaged for each fish. Error bars represent standard deviation. NS, not significant. Figure 2: Zygotic ptk7 mutants do not display vertebral patterning abnormalities but do show vertebral ‘wedging’ reminiscent of human IS. ( a – f ) Live calcein staining of ( a , b ) 4 mm, ( c , d ) 4.5 mm and ( e , f ) 6.0 mm ( a , c , e ) ptk7 heterozygote and ( b , d , f ) zygotic ptk7 (Z ptk7 ) mutant larvae. All scale bars, 0.5 mm. ( g , h ) Lateral views of caudal vertebrae from three-dimensional microCT renderings of adult ( g ) ptk7 heterozygote and ( h ) Z ptk7 mutant zebrafish. Ptk7 mutant vertebrae display a wedge-shaped morphology at the apex of curves. ( i , j ) Graphs depicting dorsal:ventral and left:right length ratios of trunk and tail vertebrae in ptk7 heterozygote ( i ; n =3) and Z ptk7 mutant ( j ; n =12) zebrafish. To characterize vertebral shape changes, we measured the length of individual thoracic and tail vertebrae along the dorsal, ventral, left and right sides. We calculated dorsal:ventral and left:right length ratios to assess possible length asymmetries in the dorso-ventral and medio-lateral planes, respectively. Horizontal dotted lines demarcate arbitrary±0.1, determined by the maximum deviation from 1 in ptk7 heterozygote controls and used to illustrate the deviation of Z ptk7 vertebrae from normal. Deviation from 1±0.1 is evident at multiple vertebrae in three dimensions along the entire length of the spine. Type 1–4 Z ptk7 mutants are grouped by point colour, and each individual fish is represented by a unique point shape and colour. The graph’s horizontal axis spans anterior (A) to posterior (P), from the first abdominal vertebrae to the last caudal vertebrae. The Weberian and caudal tail vertebrae were excluded from our analysis. ( k , l ) Maximum intensity projections (MIP) in the cranio–caudal direction from high-resolution micro-computed tomography (microCT) of ( k ) ptk7 /+ and ( l ) Z ptk7 mutant zebrafish. Dorsal is up and ventral is down. ( m ) Quantification of maximum pixel intensity corrected for background intensity to infer approximate bone density in ptk7/ + ( n =3) and Z ptk7 ( n =12) zebrafish. Maximum pixel intensities of the vertebrae were extracted from MIPs made from 10 sequential microCT slices. Three locations from trunk to tail were quantified and averaged for each fish. Error bars represent standard deviation. NS, not significant. Full size image To characterize vertebral shape changes, we measured the length of individual thoracic and tail vertebrae along the dorsal, ventral, left and right sides. We calculated dorsal:ventral and left:right length ratios to assess possible length asymmetries in the dorso-ventral and medio-lateral planes, respectively. Asymmetric or ‘wedge-shaped’ vertebral distortions were associated with the apex of spinal curves in adult fish, consistent with human IS where vertebrae become misshapen with disease progression ( Fig. 2g,h ) [33] , [34] , [35] , [36] . The affected vertebrae occurred throughout the trunk and tail with no strong positional bias ( Fig. 2i,j ). Analysis of vertebral bone density revealed no significant difference between Z ptk7 mutant and ptk7 /+ animals ( Fig. 2k–m ). To pinpoint the onset of scoliosis in mutant animals, the length and physical appearance of ptk7 /+ and Z ptk7 mutant larvae were closely monitored over the first 6 weeks of life ( Fig. 3a ). Curve onset could first be detected in Z ptk7 mutants at 8 mm standard length (~28 days post fertilization (dpf)), as fish began to exhibit mild body distortions ( n =18/23, 78%; Fig. 3e ) associated with sagittal curvature of the spine (as confirmed by microCT, Fig. 3f ). Of note, curve development correlated with the onset of a period of accelerated growth ( Fig. 3a ). By 1.2 mm standard length (~40 dpf) all Z ptk7 mutants displayed obvious axial curvatures, with some showing three-dimensional rotations ( n =5/23; Fig. 3m ) that increased in magnitude up to late juvenile stages. Curve severity did not visibly progress after sexual maturity (~3 months of age) and adult fish could be grouped into four classes (type 1–4) based on increasing magnitude of spinal curvatures ( Fig. 1c–m ) [37] . Notably, female Z ptk7 mutants demonstrated a clear bias towards severe curves (93%, n =58; Fig. 1c ). Late-onset spinal curvatures of Z ptk7 mutant zebrafish thus closely model the defining attributes of human adolescent IS. 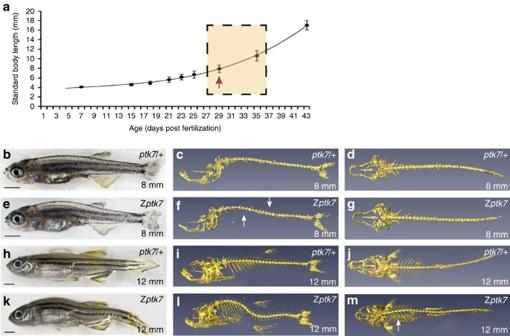Figure 3: Zygoticptk7mutants develop spinal curvatures that progress rapidly during late larval and early juvenile stages. (a) Graph depicting standard body length measurements65of Zptk7andptk7/+ larvae during the first 42 days of development (sample numbers: 6 dpf=16, 14 dpf=89, 17 dpf=72, 20 dpf=51, 22 dpf=48, 24 dpf=47, 28 dpf=48, 35 dpf=48, 42 dpf=40). Zptk7began to display axial curves at 8 mm standard body length (red arrow) and curves progress through to juvenile stages, which represents a time of accelerated growth (orange box). After 8 mm standard body length, Zptk7mutant juveniles were not included as axial curvatures prevented accurate measurements. Data points represent average body length and error bars represent standard deviation. (b–d)ptk7/+ and (e–g) Zptk7mutant zebrafish at 8 mm standard body length. (h–j)ptk7/+ and (k–m) Zptk7mutant zebrafish at 12 mm body length. Scale bars, 1 mm. (c,f,i,l) Lateral and (d,g,j,m) dorsal views of three-dimensional microCT renderings of (c,d,i,j) ptk7/+ and (f,g,l,m) Zptk7 mutants. At the time of onset, Zptk7mutants display sagittal spinal curves (arrows inf) that can increase in severity to three-dimensional scoliosis (medio-lateral deviation, arrow inm). Figure 3: Zygotic ptk7 mutants develop spinal curvatures that progress rapidly during late larval and early juvenile stages. ( a ) Graph depicting standard body length measurements [65] of Z ptk7 and ptk7 /+ larvae during the first 42 days of development (sample numbers: 6 dpf=16, 14 dpf=89, 17 dpf=72, 20 dpf=51, 22 dpf=48, 24 dpf=47, 28 dpf=48, 35 dpf=48, 42 dpf=40). Z ptk7 began to display axial curves at 8 mm standard body length (red arrow) and curves progress through to juvenile stages, which represents a time of accelerated growth (orange box). After 8 mm standard body length, Z ptk7 mutant juveniles were not included as axial curvatures prevented accurate measurements. Data points represent average body length and error bars represent standard deviation. ( b – d ) ptk7 /+ and ( e – g ) Z ptk7 mutant zebrafish at 8 mm standard body length. ( h – j ) ptk7 /+ and ( k – m ) Z ptk7 mutant zebrafish at 12 mm body length. Scale bars, 1 mm. ( c , f , i , l ) Lateral and ( d , g , j , m ) dorsal views of three-dimensional microCT renderings of ( c , d , i , j ) ptk7/+ and ( f , g , l , m ) Zptk7 mutants. At the time of onset, Z ptk7 mutants display sagittal spinal curves (arrows in f ) that can increase in severity to three-dimensional scoliosis (medio-lateral deviation, arrow in m ). Full size image A novel human PTK7 mutation disrupts Wnt signalling activity To investigate the mutational burden that PTK7 may contribute to human IS, we Sanger sequenced PTK7 coding exons of 96 human IS samples and identified four distinct missense variants ( Supplementary Table 1 ). Two missense variants were rare (<1% frequency in public databases). We genotyped the two variants, single nucleotide polymorphisms (SNPs) rs34021075 and rs34865794 in a follow-up cohort of 755 non-Hispanic white (NHW) cases and 1,392 NHW controls, but neither was significantly associated with IS independently or in combination ( Supplementary Table 2 ). Of particular interest was a novel heterozygous PTK7 sequence variant identified in a single IS patient and his father (who did not display spinal deformity). The patient, a 15-year-old male of Asian descent, presented with typical features of IS, a 49 degree right thoracic curve and no other associated clinical findings ( Fig. 4a ). His curve eventually progressed and required corrective surgery. The PTK7 missense variant occurred in exon 11, predicting a proline to alanine substitution (PTK7 P545A ) within an evolutionarily conserved residue of the sixth extracellular Ig loop. This mutation was novel, as it was not found in any public database (for example, dbSNP or the NHLBI exome variant server), nor in our in-house exome sequencing controls. The variant was also not present in 1,030 additional IS cases and 400 genotyped controls. 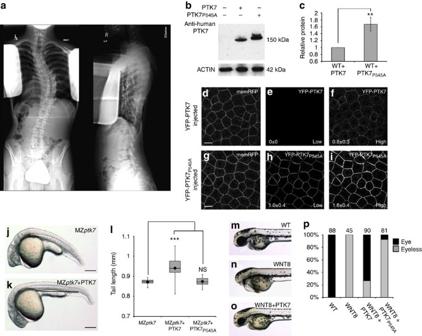Figure 4: The P545A variant affects PTK7 Wnt signalling potential. (a) Patient X-ray. (b) Human PTK7 in total cell lysates made from uninjected wild-type (WT) shield-staged zebrafish embryos, or WT embryos injected at the one-cell stage with 250 pg of eitherPTK7orPTK7P545AmRNA. Actin is used as a loading control. (c) Quantification of relative PTK7 and PTK7P545Aprotein levels (n=3, **P=0.0036). Protein levels were normalized to actin and PTK7 was set to 1. (d–i) Confocal images of the animal cap of embryos at 60% epiboly co-injected at the one-cell stage with membrane-localized monomeric red fluorescent protein (membrane RFP)70and either yellow fluorescent protein (YFP)-taggedPTK7(250 pg) orPTK7P545A(250 pg) mRNA. Scale bars, 200 μm. Co-expressed (d) membrane RFP and (e–f) YFP-PTK7 visualized at (e) low (720 V) and (f) high (920 V) intensity. Co-expressed (g) membrane RFP and (h) YFP–PTK7P545Aat low (720 V) and (g) high (920 V) intensity. Numerical values represent average membrane YFP intensity normalized to membrane RFP fluorescent intensity (lowP<0.001, highP<0.001;n=60 for each sample). At high (920 V) intensity the YFP–PTK7P545Asignal was above saturation. Lateral views of (j) MZptk7and (k) MZptk7embryos injected withPTK7(100 pg) mRNA at 24 hpf. Scale bars, 200 μm. (l) Quantification of tail length (mm) at 24 hpf measured from the base of the yolk extension to the tail tip in MZptk7mutant embryos (n=13) or MZptk7mutant embryos injected with 100 pg of eitherPTK7(n=58) orPTK7P545A(n=60) mRNA. The bottom and top of each box represent the first and third quartile, respectively; central line represents the median; bars represent the minimum and maximum tail lengths. PTK7 rescues tail extension defects in MZptk7(***P<0.0001, Student’st-test).PTK7P545AmRNA (100 pg) has no effect on axial extension, suggesting reduced PCP signalling activity. (m–p) Over-expression ofwnt8disrupts central nervous system pattern, demonstrated by loss of eyes and reduced forebrain. Lateral views of 48 hpf (m) WT embryos and embryos injected with (n)wnt8(10 pg) or (o)wnt8(10 pg) plusPTK7(250 pg) mRNA. Co-injection ofPTK7(250 pg) mRNA rescueswnt8-induced phenotypes. (p) Quantification of phenotypes observed with injection ofwnt8(10 pg) mRNA, and with co-injection ofwnt8withPTK7(250 pg) orPTK7P545A(250 pg) mRNA. Embryos were scored as being ‘eyeless’ only if the eye was completely absent. PTK7P545Ais less efficient than PTK7 at rescuing wnt8-induced phenotypes, indicating reduced activity in Wnt/β-catenin inhibition. NS, not significant. Figure 4: The P545A variant affects PTK7 Wnt signalling potential. ( a ) Patient X-ray. ( b ) Human PTK7 in total cell lysates made from uninjected wild-type (WT) shield-staged zebrafish embryos, or WT embryos injected at the one-cell stage with 250 pg of either PTK7 or PTK7 P545A mRNA. Actin is used as a loading control. ( c ) Quantification of relative PTK7 and PTK7 P545A protein levels ( n =3, ** P =0.0036). Protein levels were normalized to actin and PTK7 was set to 1. ( d – i ) Confocal images of the animal cap of embryos at 60% epiboly co-injected at the one-cell stage with membrane-localized monomeric red fluorescent protein (membrane RFP) [70] and either yellow fluorescent protein (YFP)-tagged PTK7 (250 pg) or PTK7 P545A (250 pg) mRNA. Scale bars, 200 μm. Co-expressed ( d ) membrane RFP and ( e – f ) YFP-PTK7 visualized at ( e ) low (720 V) and ( f ) high (920 V) intensity. Co-expressed ( g ) membrane RFP and ( h ) YFP–PTK7 P545A at low (720 V) and ( g ) high (920 V) intensity. Numerical values represent average membrane YFP intensity normalized to membrane RFP fluorescent intensity (low P <0.001, high P <0.001; n =60 for each sample). At high (920 V) intensity the YFP–PTK7 P545A signal was above saturation. Lateral views of ( j ) MZ ptk7 and ( k ) MZ ptk7 embryos injected with PTK7 (100 pg) mRNA at 24 hpf. Scale bars, 200 μm. ( l ) Quantification of tail length (mm) at 24 hpf measured from the base of the yolk extension to the tail tip in MZ ptk7 mutant embryos ( n =13) or MZ ptk7 mutant embryos injected with 100 pg of either PTK7 ( n =58) or PTK7 P545A ( n =60) mRNA. The bottom and top of each box represent the first and third quartile, respectively; central line represents the median; bars represent the minimum and maximum tail lengths. PTK7 rescues tail extension defects in MZ ptk7 (*** P <0.0001, Student’s t -test). PTK7 P545A mRNA (100 pg) has no effect on axial extension, suggesting reduced PCP signalling activity. ( m – p ) Over-expression of wnt8 disrupts central nervous system pattern, demonstrated by loss of eyes and reduced forebrain. Lateral views of 48 hpf ( m ) WT embryos and embryos injected with ( n ) wnt8 (10 pg) or ( o ) wnt8 (10 pg) plus PTK7 (250 pg) mRNA. Co-injection of PTK7 (250 pg) mRNA rescues wnt8 -induced phenotypes. ( p ) Quantification of phenotypes observed with injection of wnt8 (10 pg) mRNA, and with co-injection of wnt8 with PTK7 (250 pg) or PTK7 P545A (250 pg) mRNA. Embryos were scored as being ‘eyeless’ only if the eye was completely absent. PTK7 P545A is less efficient than PTK7 at rescuing wnt8-induced phenotypes, indicating reduced activity in Wnt/β-catenin inhibition. NS, not significant. Full size image We have previously shown that the extracellular domain of zebrafish Ptk7 is essential for its role in Wnt signal transduction [24] . To determine the functional consequence of the PTK7 P545A mutation in vivo , we compared the activity of both wild-type (WT) and mutant isoforms following messenger RNA (mRNA) injection into zebrafish embryos. In western blots of whole embryo lysates, PTK7 P545A accumulated at greater levels than WT, suggesting increased stability and/or differential modification of PTK7 P545A protein ( Fig. 4b,c ; Supplementary Fig. 1 ). Similarly, membrane localization of yellow fluorescent protein-tagged PTK7 P545A was dramatically increased compared with WT PTK7 (normalized to co-injected membrane-localized monomeric red fluorescent protein, Fig. 4d–i ), suggesting that the P545A variation affects trafficking and/or turnover of PTK7 at the plasma membrane. Injection of full length zebrafish ptk7 mRNA into one-cell staged MZ ptk7 mutant embryos can rescue patterning and morphogenesis defects associated with dysregulated Wnt signalling [24] . To determine how the P545A variant affects PTK7 function, we performed similar rescue assays using human PTK7 mRNA. Strikingly, although injection of 100 pg of WT PTK7 mRNA into one-cell staged embryos significantly rescued PCP-mediated axial extension defects of MZ ptk7 mutants, injection of equal amounts of PTK7 P545A mRNA had no effect ( Fig. 4j–l ). This data indicates that the P545A PTK7 mutation disrupts its non-canonical Wnt/PCP signalling activity. Similarly, injection of WT PTK7 mRNA could rescue central nervous system patterning defects caused by wnt8 overexpression (loss of eyes and reduced forebrain at 36 hours post fertilization (hpf)). However, injection of equal amounts of PTK7 P545A mRNA failed to rescue, indicating that the P545A variant also significantly disrupts PTK7 function in inhibiting canonical Wnt/β-catenin activity ( Fig. 4m–p ). Together, these data suggest that the P545A variant is a hypomorphic allele of PTK7 . Although pathogenesis of the PTK7 P545A variant in IS remains uncertain, our results highlight the utility of the zebrafish model for investigating the functional consequence of IS-associated PTK7 mutations in vivo . MZ ptk7 mutants develop CVMs To further investigate the function of Ptk7 in spine morphogenesis, we analyzed vertebrae formation in MZ ptk7 mutant fish, which demonstrate loss-of-gene function at the earliest stages of embryogenesis [24] . Strikingly, unlike Z ptk7 mutants, MZ ptk7 larvae displayed severe congenital vertebral abnormalities at 4.8 mm standard length, including missing or smaller vertebral segments, hemivertebrae and/or vertebral fusions ( Fig. 5a ). 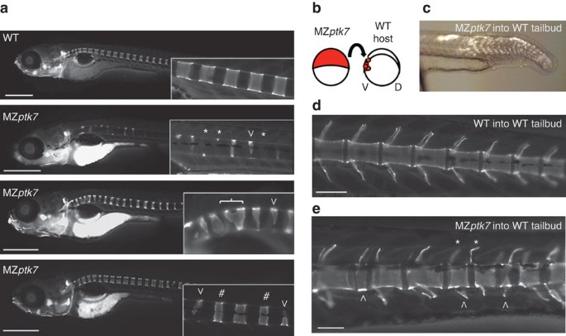Figure 5: Maternal-zygoticptk7mutant zebrafish display congenital vertebral abnormalities. (a) Live calcein staining of WT and MZptk7larvae at wild-type 4.8 mm standard length. Insets highlight representative vertebral malformations present in MZptk7mutants. Asterisks and arrowheads highlight missing and hemivertebrae, respectively. Bracket highlights vertebral fusions. Hashtags highlight smaller vertebral segments. Scale bars, 0.5 mm. (b) Transplant strategy used to generate chimeric zebrafish for late larval-stage analysis. MZptk7cells were labelled with rhodamine red and transplanted at 4 hpf into the ventral marginal zone (fated to become the embryonic tail bud) of shield stage (6 hpf) unlabelled wild-type embryos.38(c) Lateral view of 24 hpf chimeric embryo with fluorescently labelled MZptk7mutant cells present in the tail of an otherwise wild-type embryo. (d) Lateral views of caudal vertebrae in a control chimeric larvae and (e) in an MZptk7chimeric larva at 6.2–6.5 mm standard length. MZptk7cell contribution to the tail leads to vertebral malformations in otherwise wild-type larvae. Arrowheads highlight multiple abnormal vertebrae. Asterisks highlight mislocated vertebral spines (sclerotome derived). Scale bars, 100 μm. Figure 5: Maternal-zygotic ptk7 mutant zebrafish display congenital vertebral abnormalities. ( a ) Live calcein staining of WT and MZ ptk7 larvae at wild-type 4.8 mm standard length. Insets highlight representative vertebral malformations present in MZ ptk7 mutants. Asterisks and arrowheads highlight missing and hemivertebrae, respectively. Bracket highlights vertebral fusions. Hashtags highlight smaller vertebral segments. Scale bars, 0.5 mm. ( b ) Transplant strategy used to generate chimeric zebrafish for late larval-stage analysis. MZ ptk7 cells were labelled with rhodamine red and transplanted at 4 hpf into the ventral marginal zone (fated to become the embryonic tail bud) of shield stage (6 hpf) unlabelled wild-type embryos. [38] ( c ) Lateral view of 24 hpf chimeric embryo with fluorescently labelled MZ ptk7 mutant cells present in the tail of an otherwise wild-type embryo. ( d ) Lateral views of caudal vertebrae in a control chimeric larvae and ( e ) in an MZ ptk7 chimeric larva at 6.2–6.5 mm standard length. MZ ptk7 cell contribution to the tail leads to vertebral malformations in otherwise wild-type larvae. Arrowheads highlight multiple abnormal vertebrae. Asterisks highlight mislocated vertebral spines (sclerotome derived). Scale bars, 100 μm. Full size image The majority of MZ ptk7 mutant larvae die before their vertebrae are fully mineralized. Therefore, to determine the role for Ptk7 in later aspects of vertebral patterning, we generated genetic chimeras. Briefly, 100–200 MZ ptk7 mutant cells were transplanted into the ventral domain of shield stage WT embryos ( Fig. 5b ), which is fated to contribute to multiple lineages of the trunk and tail, including spinal cord and vertebrae [38] . We screened host embryos at 24 hpf for significant MZ ptk7 cell contribution within the embryonic tail ( Fig. 5c ), and raised chimeric zebrafish to larval stages. At 6.2–6.5 mm standard length, calcein staining revealed multiple vertebral malformations in ~27% of chimeric larvae, including smaller and irregularly shaped vertebral bodies and mislocated sclerotome-derived vertebral spines ( n =8/30, Fig. 5e ). These results indicate that chimeric loss of ptk7 in the tail is sufficient to disrupt vertebral patterning at later stages of development. Transplantation of WT cells into a WT embryonic tail bud did not affect vertebral patterning ( n =42, Fig. 5d ), indicating that observed phenotypes were specific to loss of ptk7 . CVMs are a hallmark of CS, and are thought to arise during early embryogenesis as a result of abnormal segmentation and somite formation [3] , [39] . To determine whether segmentation is disrupted in MZ ptk7 mutant embryos, we performed in situ hybridization of her7 and dlc (direct reporters of the Notch segmentation mechanism and nascent somite differentiation) [40] within the PSM of 18–20 somite-staged MZ ptk7 mutant embryos, looking for possible irregularities in gene expression. The PSM domain was broader and expanded relative to total body length in MZ ptk7 mutants, consistent with a role for Ptk7 in tail-bud patterning and morphogenesis [24] . Of note, although her7 ( n =24) and dlc ( n =18) gene expression appeared to oscillate normally in MZ ptk7 mutant embryos ( Fig. 6a,b ), occasional irregularities in the symmetry of gene expression were observed ( n =9/24 in her7 ; Fig. 6a ), indicating possible defects in somite patterning. Strikingly, myoD and Xirp2a (ref. 41 ) expression analysis revealed severe defects in the regular morphology and spacing of the somites in MZ ptk7 mutants, as well as somite fusions ( Fig. 6c–f ). Visualization of pax9 gene expression also revealed abnormalities in the regular pattern of sclerotome in MZ ptk7 mutants ( Fig. 6g,h ), consistent with abnormal somite patterning. 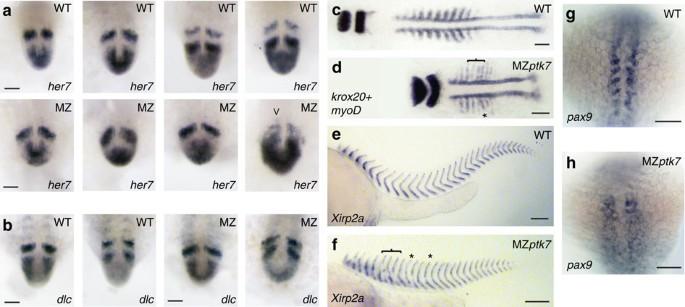Figure 6: Maternal-zygoticptk7mutant embryos display segmentation defects. (a,b) Whole-mountin situhybridization (WISH) of somite patterning gene expression at the 18–20 somite stage. All images are posterior views with the embryonic tail bud pointing towards the bottom of the field of view. WT and MZptk7mutant embryos stained for (a)her7, (b)dlcexpression. The expression domains of these markers is expanded within MZptk7mutants consistent with PSM morphogenetic defects24. Arrowhead inahighlights anterior domain asymmetry in one MZptk7mutant embryo. Scale bars, 50 μm. (c,d)myoD(somite) staining in (c) WT and (d) MZptk7embryos to visualize segmentation during somitogenesis. MZptk7display defects in the regular spacing and morphology of the somites at this stage. Scale bars, 100 μm. (e,f) Lateral view of WISH forXirp2aexpression to mark somite boarders41in (e) WT and (f) MZptk7mutant embryos at 40 hpf. The horizontal brackets and asterisks highlight examples of somite fusions. Defects in the shape and size of the somites are also apparent in MZptk7mutants. Scale bars, 100 μm. (g,h)pax9expression in (g) WT and (h) MZptk7mutant embryos to visualize sclerotome. Scale bars, 100 μm. Figure 6: Maternal-zygotic ptk7 mutant embryos display segmentation defects. ( a , b ) Whole-mount in situ hybridization (WISH) of somite patterning gene expression at the 18–20 somite stage. All images are posterior views with the embryonic tail bud pointing towards the bottom of the field of view. WT and MZ ptk7 mutant embryos stained for ( a ) her7 , ( b ) dlc expression. The expression domains of these markers is expanded within MZ ptk7 mutants consistent with PSM morphogenetic defects [24] . Arrowhead in a highlights anterior domain asymmetry in one MZ ptk7 mutant embryo. Scale bars, 50 μm. ( c , d ) myoD (somite) staining in ( c ) WT and ( d ) MZ ptk7 embryos to visualize segmentation during somitogenesis. MZ ptk7 display defects in the regular spacing and morphology of the somites at this stage. Scale bars, 100 μm. ( e , f ) Lateral view of WISH for Xirp2a expression to mark somite boarders [41] in ( e ) WT and ( f ) MZ ptk7 mutant embryos at 40 hpf. The horizontal brackets and asterisks highlight examples of somite fusions. Defects in the shape and size of the somites are also apparent in MZ ptk7 mutants. Scale bars, 100 μm. ( g , h ) pax9 expression in ( g ) WT and ( h ) MZ ptk7 mutant embryos to visualize sclerotome. Scale bars, 100 μm. Full size image Importantly, we did not observe segmentation defects in Z ptk7 mutant embryos ( Fig. 7 ). This indicates that maternally derived ptk7 gene product (present at the one-cell stage) is sufficient to rescue somitogenesis in Z ptk7 mutant zebrafish. More importantly, since maternal ptk7 is not expected to persist beyond early embryonic stages [42] , our data strongly suggest that CVMs observed in MZ ptk7 mutants are directly linked to early embryonic defects in patterning and morphogenesis. 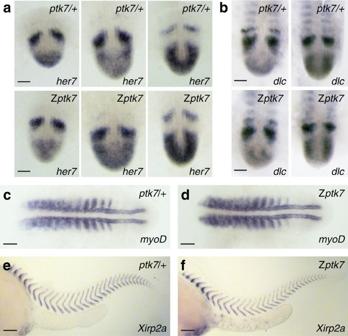Figure 7: Zygoticptk7mutant embryos do not display segmentation defects. (a)her7and (b)dlcexpression inptk7/+ and Zptk7mutant embryos at the 18–20 somite stage. No obvious defects in somitogenesis exist in Zptk7mutant embryos. Scale bars, 50 μm. (c,d)myoD(somite) staining in (c)ptk7/+ and (d) Zptk7embryos to visualize segmentation during somitogenesis. Scale bars, 100 μm. (e,f) Lateral view of WISH forXirp2aexpression to mark somite boarders41in (e)ptk7/+ and (f) Zptk7mutant embryos at 40 hpf. Zptk7do not display defects in embryonic segmentation, indicating maternal rescue of the axial patterning defect. Scale bars, 100 μm. Figure 7: Zygotic ptk7 mutant embryos do not display segmentation defects. ( a ) her7 and ( b ) dlc expression in ptk7 /+ and Z ptk7 mutant embryos at the 18–20 somite stage. No obvious defects in somitogenesis exist in Z ptk7 mutant embryos. Scale bars, 50 μm. ( c , d ) myoD (somite) staining in ( c ) ptk7 /+ and ( d ) Z ptk7 embryos to visualize segmentation during somitogenesis. Scale bars, 100 μm. ( e , f ) Lateral view of WISH for Xirp2a expression to mark somite boarders [41] in ( e ) ptk7 /+ and ( f ) Z ptk7 mutant embryos at 40 hpf. Z ptk7 do not display defects in embryonic segmentation, indicating maternal rescue of the axial patterning defect. Scale bars, 100 μm. Full size image Abnormal PCP disrupts segmentation and vertebral patterning It is well-understood that Wnt/β-catenin signalling within the PSM is required for axial segmentation [43] , [44] , [45] . Since MZ ptk7 display activated Wnt/β-catenin signalling in the embryonic tailbud [24] , we treated WT embryos with the canonical Wnt/β-catenin agonists LiCl [46] or 6-bromoindirubin-3′-oxime (BIO) [47] throughout somitogenesis to determine the consequence on segmentation and vertebral patterning. Both regiments resulted in somite boundary defects at 40 hpf ( Fig. 8a,b ) as well as smaller and/or fused vertebral segments at larval stages ( Fig. 8c,d ), which closely phenocopied MZ ptk7 mutant animals. 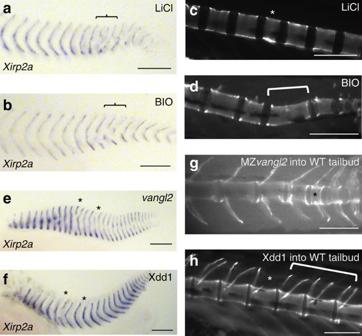Figure 8: Abnormal non-canonical Wnt/PCP or canonical Wnt/β-catenin signalling lead to defects in embryonic segmentation and to subsequent vertebral abnormalities. (a,b) Lateral view of whole-mountin situhybridization (WISH) at 40 hpf forXirp2aexpression to mark somite boundaries41in embryos treated during mid-somitogenesis (10 somites—24 hpf) with canonical Wnt/β-catenin agonist (a) 0.1 M LiCl or (b) 10 μM BIO. Brackets highlight segmental fusions. Scale bars, 100 μm. (c,d) Lateral views of live calcein staining in 5–6 mm standard length wild-type larvae treated throughout somitogenesis (bud stage—24 hpf) with (c) 10 μM LiCl or (d) 1 μM BIO. Scale bars, 100 μm. Activation of canonical Wnt/β-catenin signalling leads to vertebral abnormalities phenotypically similar to MZptk7loss-of-function including smaller vertebral segments (white asterisk) and/or vertebral fusions (white bracket). (e,f) Lateral view of WISH forXirp2aexpression to mark somite boundaries41in (e)vangl2mutant embryos and (f) embryos injected withXdd1(150 pg) mRNA. Asterisks highlight examples of somite fusions. Scale bars, 100 μm. Disruption of non-canonical Wnt/PCP signalling results in defects in embryonic segmentation. (g,h) Lateral views of live calcein staining in wild-type host larvae at 6.2–6.5 mm standard length that were transplanted with (g) MZvangl2mutant cells or (h) cells injected withXdd1(150 pg) mRNA. Transplantation was performed to bypass early lethality of MZvangl2mutants orXdd1overexpression. Donor cells were transplanted into the ventral margin (future tail bud) of wild-type hosts.38Scale bars, 100 μm. Disruption of non-canonical Wnt/PCP signalling in the tail-bud region results in vertebral abnormalities phenotypically similar to MZptk7loss-of-function, including smaller vertebral segments (black asterisk), asymmetric (white bracket) or mislocated vertebral arches (white asterisk). Figure 8: Abnormal non-canonical Wnt/PCP or canonical Wnt/β-catenin signalling lead to defects in embryonic segmentation and to subsequent vertebral abnormalities. ( a , b ) Lateral view of whole-mount in situ hybridization (WISH) at 40 hpf for Xirp2a expression to mark somite boundaries [41] in embryos treated during mid-somitogenesis (10 somites—24 hpf) with canonical Wnt/β-catenin agonist ( a ) 0.1 M LiCl or ( b ) 10 μM BIO. Brackets highlight segmental fusions. Scale bars, 100 μm. ( c , d ) Lateral views of live calcein staining in 5–6 mm standard length wild-type larvae treated throughout somitogenesis (bud stage—24 hpf) with ( c ) 10 μM LiCl or ( d ) 1 μM BIO. Scale bars, 100 μm. Activation of canonical Wnt/β-catenin signalling leads to vertebral abnormalities phenotypically similar to MZ ptk7 loss-of-function including smaller vertebral segments (white asterisk) and/or vertebral fusions (white bracket). ( e , f ) Lateral view of WISH for Xirp2a expression to mark somite boundaries [41] in ( e ) vangl2 mutant embryos and ( f ) embryos injected with Xdd1 (150 pg) mRNA. Asterisks highlight examples of somite fusions. Scale bars, 100 μm. Disruption of non-canonical Wnt/PCP signalling results in defects in embryonic segmentation. ( g , h ) Lateral views of live calcein staining in wild-type host larvae at 6.2–6.5 mm standard length that were transplanted with ( g ) MZ vangl2 mutant cells or ( h ) cells injected with Xdd1 (150 pg) mRNA. Transplantation was performed to bypass early lethality of MZ vangl2 mutants or Xdd1 overexpression. Donor cells were transplanted into the ventral margin (future tail bud) of wild-type hosts. [38] Scale bars, 100 μm. Disruption of non-canonical Wnt/PCP signalling in the tail-bud region results in vertebral abnormalities phenotypically similar to MZ ptk7 loss-of-function, including smaller vertebral segments (black asterisk), asymmetric (white bracket) or mislocated vertebral arches (white asterisk). Full size image Ptk7 is also required for non-canonical Wnt/PCP signalling. Although previous studies suggest that somite segmentation is unaffected in PCP mutant zebrafish [48] , our analysis of 40 hpf vangl2 mutant embryos (also known as trilobite , deficient for a core and specific regulator of PCP signal transduction) [49] revealed segmentation defects that were similar to MZ ptk7 animals ( n =8/8, Fig. 8e ). Furthermore, injection of Xdd1 mRNA (a dominant-negative Dishevelled construct that specifically disrupts PCP) [50] produced similar phenotypes ( n =15/18; Fig. 8f ). v angl2 mutant and Xdd1 -injected embryos both die before mineralized vertebrae can be visualized. Therefore, to determine the consequence of abnormal PCP on vertebrae formation, we transplanted mutant cells into the tail bud of WT host embryos and scored vertebral development at larval stages. Both MZ vangl2 mutant and Xdd1 -injected chimeras ( n =8/12 and 9/16, respectively) demonstrated malformed vertebral centra and/or vertebral arches analogous to those observed in MZ ptk7 mutant larvae ( Fig. 8g,h ). Therefore, our data indicates that defects in both PCP and Wnt/β-catenin signalling can contribute to segmentation defects and vertebral malformations, suggesting novel genetic and developmental etiologies of CS. Ptk7 is a key regulator of canonical Wnt/β-catenin and non-canonical Wnt/PCP signalling activity and is required for vertebrate embryonic patterning and morphogenesis [24] , [26] , [28] . However, maternal rescue of early developmental abnormalities in Z ptk7 mutant zebrafish reveals an important later requirement in spine morphogenesis. As demonstrated, Z ptk7 mutant zebrafish develop fully penetrant, late-onset, three-dimensional curvatures of the spine at late larval/early juvenile stages—a period associated with accelerated growth. Females demonstrate a strong bias for severe curves, which can progress in magnitude until sexual maturity. Z ptk7 mutant phenotypes thus closely model defining attributes of human adolescent IS. As stated, while IS has been difficult to model in more conventional lab animals, spinal curvature is a common phenotype among fish [23] , [51] . It has been postulated that cranial-to-caudal spinal loads generated by teleost locomotion mimic biomechanical forces and spinal loads resulting from human upright posture—a contributing factor in IS development and progression. Indeed a number of heritable late-onset scoliosis models have been reported in fish [37] , [52] , although genetic lesions responsible for these phenotypes have not yet been identified. Z ptk7 mutant zebrafish thus represent the first genetically defined developmental model of human IS. A comprehensive investigation into the contribution of PTK7 mutations in human IS is yet to be performed. However, conservation of Ptk7 function between zebrafish and humans allowed us to directly assess the consequence of a novel PTK7 sequence variant identified in a single IS patient. Remarkably, the PTK7 P545A allele disrupts both canonical Wnt/β-catenin and non-canonical Wnt/PCP signalling activity, consistent with a role for dysregulated Wnt signalling in IS. Ptk7 is known to interact with Wnt ligands, Frizzled 7 and LRP6 co-receptors [28] , [53] , [54] , suggesting that PTK7 is a functional component of the Wnt receptor complex. Since receptor complex endocytosis is an essential component of both Wnt/PCP and Wnt/β-catenin signal activation [55] , [56] , [57] , observed increases in PTK7 P545A plasma membrane localization suggest that the P545A variant could disrupt Wnt signalling by altering complex trafficking. Pathogenesis of the PTK7 P545A variant in IS remains to be determined. Despite strong conservation of the PTK7 P545 residue among mammals, it is not conserved in zebrafish confounding requisite ‘knock-in’ studies. Nevertheless, our functional and genetic results suggest that PTK7 and other Wnt signalling pathway members warrant further re-sequencing in large IS cohorts. Unexpectedly, maternal-zygotic ptk7 mutant larvae develop vertebral malformations typically associated with CS. Although canonical Wnt/β-catenin signalling activity has previously been implicated in segmentation [3] , [44] , we demonstrate that non-canonical Wnt/PCP defects may also contribute to vertebral malformations and CS pathogenesis. Previous studies have correlated PCP-related axial defects (neural tube disorders) with CVMs [58] , [59] . Our analysis of Vangl2 mutant embryos and chimeras clearly show a direct role for PCP in segmentation and vertebral patterning. Of interest, MZ ptk7 mutants did not exhibit severe misregulation or asymmetries in somite gene patterning that are typically observed following disruption of core segmentation genes [60] , [61] , [62] . However, mild abnormalities/asymmetries in PSM domain morphology may be sufficient to cause the irregular somite defects observed during later stages of development. Consequently, the MZ ptk7 mutant phenotype may be more reminiscent of non-syndromic mild or moderate cases of CS where individuals display relatively few CVMs at irregular locations along the length of the spine [3] . To summarize, depending on the timing of loss of Ptk7 function, MZ ptk7 and Z ptk7 mutant zebrafish develop distinct spinal deformities that model CS and IS, respectively ( Fig. 9 ). Although CS and IS have long been classified as distinct and separate disorders, a number of independent studies have reported an increased incidence of IS among the family members of CS subjects [5] , [63] , [64] . Our study thus provides further evidence that congenital and idiopathic forms of scoliosis may share a common genetic basis. 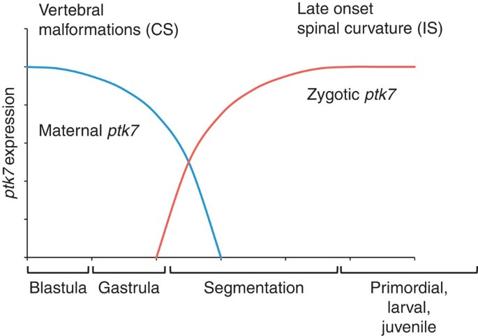Figure 9:Ptk7mutants model CS or IS depending on timing of gene loss-of-function. Maternalptk7is deposited in the egg and drives early development including Ptk7-dependent morphogenesis24and segmentation. Loss of maternal (solid blue line) and zygoticptk7(solid red line) leads to segmentation defects and vertebral malformations that recapitulate human CS. Zygotic loss ofptk7leads to late-onset spinal curvature with no underlying vertebral malformations that recapitulate human IS. Figure 9: Ptk7 mutants model CS or IS depending on timing of gene loss-of-function. Maternal ptk7 is deposited in the egg and drives early development including Ptk7-dependent morphogenesis [24] and segmentation. Loss of maternal (solid blue line) and zygotic ptk7 (solid red line) leads to segmentation defects and vertebral malformations that recapitulate human CS. Zygotic loss of ptk7 leads to late-onset spinal curvature with no underlying vertebral malformations that recapitulate human IS. Full size image The biological relationship (if any) between CS and IS is yet to be determined. Although somite and vertebral patterning defects are not observed in Z ptk7 mutant embryos, it remains possible that subtle defects in segmentation may be later accentuated by additional genetic or environmental cues. Alternatively, the underlying cause of IS may be completely distinct from CS. Ptk7, Wnt/PCP or Wnt/β-catenin signalling have not previously been associated with human IS. However, since the genetics, biomechanics and physiology underlying zebrafish and human development are conserved, shared biological mechanisms underlying spinal curve progression are likely. Zebrafish ptk7 mutant models thus present unique opportunities for investigating the aetiology and pathogenesis of IS and CS, and promise to yield fundamental insights into the developmental, cellular and molecular origins of disease. Zebrafish strains Established zebrafish husbandry protocols were adhered to and all protocols were performed in accordance with Canadian Council on Animal Care (CCAC) guidelines. MZ ptk7 and Z ptk7 ( hsc9 ) were generated as previously described [24] . The vangl2 mutant allele tri(tk50f) contains a deletion in the vangl2 coding sequence [49] . Fish were staged based on standard body length, except in the case of MZ ptk7 mutant larvae, which were staged based on external anatomy and vital staining [65] . Alizarin red Adult zebrafish were fixed for 1 week in 4% paraformaldehyde at 4 °C followed by two, 1 h washes with phosphate-buffered saline with 0.1% Tween 20 (PBST). Fish were stained with 0.01% Alizarin red (Sigma) in 1% KOH for 1 week and washed in PBST for 3 days (1 wash/day) Tissues were cleared in 0.5% trypsin digestion for 1 day followed by multiple washes with PBST. The skin was manually removed and the skeleton was imaged on a Leica MZ16 dissecting scope using AxioVision (Zeiss) software. Calcein staining Zebrafish larvae were incubated in 0.2% Calcein (Sigma), pH 7.5 for 15 min and washed twice in system water. Larvae were immobilized using 0.003% Tricaine (Sigma) and mounted in 3% methyl cellulose. Imaging was performed on an Axio Imager.M1 (Zeiss) compound microscope. MicroCT Adult zebrafish were fixed in 10% neutral-buffered formalin for 1 week and mounted in 1% low-melt agarose (Sigma) in a plastic vial. Specimens were scanned for 1 h using SkyScan1172 high resolution Micro-CTanner (Bruker micro-CT, Belgium) with the X-ray power at 45 kVp and 218 μA. All three-dimensional Micro-CT data sets were reconstructed with 18 μm isotropic resolution. The images were then analyzed using Amira software (TGS Inc., Berlin, Germany) Plasmids and embryo microinjections WT human PTK7 was cloned from MGC clone:30347652 using primers: forward 5′- GGGGACAAGTTTGTACAAAAAAGCAGGCTTCGCCACCATGGGAGCTGCGCGGGGATC -3′ and reverse 5′- GGGACCACTTTGTACAAGAAAGCTGGGTGTCACGGCTTGCTGTCCACGGTG -3′. PTK7 P545A was cloned a in two fragments using primers: forward1 5′- ATGGGAGCTGCGCGGGGATC -3′, reverse1 5′- CACTCTGCGAGGCTGCTC -3′, and forward2 5′- GCAGAGTGGGTGACAGACAA -3′, reverse2 5′ TCACGGCTTGCTGTCCACGGTG 3′ and assembled by PCR (10 cycles of annealing and extension without primers followed by 30 cycles using WT human PTK7 forward and reverse primers). Both PTK7 and PTK7 P545A were inserted into pCS2+ expression vectors (plasmid 22423: pCSDEST, ADDGENE) using Gateway technology (Invitrogen). All mRNA was transcribed using the mMESSAGE mMACHINE System (Ambion) and was injected at the one-cell stage. PTK7 variant discovery in human IS samples All research subjects included in the PTK7 re-sequencing study provided written informed consent to participate as approved by the University of Texas Southwestern Medical Center Institutional Review Board. Twenty coding exons of PTK7 were PCR amplified from 96 IS samples as described in the text and sequenced by the Sanger method (oligonucleotide primer sequences and PCR conditions available on request). This identified four nonsynonymous changes. Two highly conserved nonsynonymous SNPs, SNPs rs34021075 and rs34865794, were genotyped by Taqman assay in 736 IS NHW cases and 740 NHW controls and tested for allelic association with IS. Embryonic transplants MZ ptk7 , MZ vangl2 or Xdd1mRNA-injected cells were labelled with rhodamine dextran (red 10,000 MW, Sigma) by injections at the one-cell stage. Labelled cells were transplanted from sphere (4 hpf) stage embryos into the ventral margin of unlabelled WT hosts at shield stage (6 hpf) as previously described [38] . Embryos were screened at 24 hpf on an Axio Imager.M1 (Zeiss) compound microscope and embryos containing significant rhodamine-labelled cells (mutant/Xdd1 cells) in the embryonic tail were grown to larval stages. Whole-mount in situ hybridization (WISH) MyoD (ref. 66 ) , krox20 (ref. 67 ) , her7 (ref. 68 ), and dlc (ref. 40 ) plasmids were obtained. Ripply1 and Xirp2a were cloned from an embryonic complementary DNA library made from total RNA using oligo(dT) 12–18 primer (Invitrogen) and SuperscriptII reverse transcriptase (Invitrogen) as per manufacturer’s instructions. The following primers were used: ripply1 forward 5′- GGGACAAGTTTGTACAAAAAGCAGGCTTCATGAATTCTGTGTGCTTTGCCA -3′, reverse 5′- GGGGACCACTTTGTACAAGAAAGCTGGGTGGTTGAAAGCTGTGAAGTGACT -3′, and Xirp2a forward 5′- GGGGACAAGTTTGTACAAAAAAGCAGGCTTCAGAGAGCATCCAGGCCACTA -3′, reverse 5′- GGGGACCACTTTGTACAAGAAAGCTGGGTGGGCCACACGACTGCAATTTT -3′. PCR products were inserted into pDONR221 vectors (Invitrogen) using Gateway technology (Invitrogen) and linearized using Apa1 restriction endonuclease. All antisense RNA probes were prepared by in vitro transcription (DIG RNA Labeling Kit, Roche) in the presence of digoxigenin-11-UTP from linearized DNA templates. Embryos were either fixed and flat mounted in 80% glycerol or cleared in 100% methanol, mounted in benzylbenzoate:benzylalcohol (2:1) and imaged on an Axio Imager.M1 (Zeiss) compound microscope. Drug treatment Embryos were incubated in 10 μM LiCl (Sigma) or 10 μM BIO (Sigma) from bud stage (10 hpf) until 24 hpf, washed in system water and grown to larval stages for vertebrae analysis. Embryos were incubated in 0.1 M LiCl or 100 μM BIO from late somite stages until 24 hpf, washed in system water and fixed in 4% paraformaldehyde for WISH. Western blot analysis Zebrafish embryos were deyolked [69] , followed by lysis in 1% NP-40 protein lysis buffer. Protein was denatured using β-mercaptoethanol buffer at 95 °C for 10 min, and separated on an 8% SDS–PAGE gel. PTK7 was detected using goat anti-human PTK7 antibody (LSBio) and mouse anti-actin (Sigma) was used as a loading control. Confocal imaging Live embryos were immobilized on a coverslip in 1% agarose, and imaged using a Zeiss LSM 710 microscope. Z-stacks were collected and processed using ImageJ software. How to cite this article: Hayes, M. et al . ptk7 mutant zebrafish models of congenital and idiopathic scoliosis implicate dysregulated Wnt signalling in disease. Nat. Commun. 5:4777 doi: 10.1038/ncomms5777 (2014).